A source of isotopically light organic carbon in a low-pH anoxic marine zone Geochemical and stable isotope measurements in the anoxic marine zone (AMZ) off northern Chile during periods of contrasting oceanographic conditions indicate that microbial processes mediating sulfur and nitrogen cycling exert a significant control on the carbonate chemistry (pH, A T , DIC and p CO 2 ) of this region. Here we show that in 2015, a large isotopic fractionation between DIC and POC, a DIC and N deficit in AMZ waters indicate the predominance of in situ dark carbon fixation by sulfur-driven autotrophic denitrification in addition to anammox. In 2018, however, the fractionation between DIC and POC was significantly lower, while the total alkalinity increased in the low-pH AMZ core, suggesting a predominance of heterotrophic processes. An isotope mass-balance model demonstrates that variations in the rates of sulfur- and nitrogen-mediated carbon fixation in AMZ waters contribute ~7–35% of the POC exported to deeper waters. Thus, dark carbon fixation should be included in assessments of future changes in carbon cycling and carbonate chemistry due to AMZ expansion. Dissolved oxygen plays a key role in shaping the structure of marine ecosystems, the spatial and temporal distribution of marine organisms [1] , and regulates both metabolic and biogeochemical processes [2] . Since oxygen (O 2 ) is slowly depleted in the ocean with depth, in some regions this leads to the formation of steady-state O 2 -deficient intermediate layers commonly known as oxygen minimum zones (OMZs) [3] , [4] . O 2 varies geographically among OMZs, but it generally falls below <20 μmol kg −1 [5] . Marine time series indicate a substantial shoaling of the upper OMZ boundary over the past decades along several eastern boundary-current systems, such as the Subarctic Pacific [6] , the eastern equatorial region [7] , and the northeast Pacific Ocean [8] . Notably, newly developed oxygen sensors [9] have demonstrated that O 2 can fall below sensor-specific detection limits (~3 nmol L −1 ) within a significant fraction of OMZ waters. Due to their extreme oxygen-depletion, OMZs like the one along the eastern tropical South Pacific (ETSP) coast off Peru and Chile have been recently redefined as anoxic marine zones (AMZs) [10] . AMZs are often distinguished from OMZs by the accumulation of nitrite, which typically occurs when O 2 falls below the nanomolar detection limit [10] . In these anoxic zones, nitrate- and sulfate-reducing bacteria, as well as methanotrophic and canonical denitrifying bacteria dominate heterotrophic processes [10] , [11] . The combination of microbially mediated remineralization process, which consumes O 2 and produces dissolved inorganic carbon (DIC), in addition to weak ventilation, leads to the establishment and persistence of O 2 -depleted waters. Organic carbon oxidation in AMZ waters is driven by microorganisms able to utilize alternative electron acceptors, which results in excess CO 2 and lower pH (< 7.8) [12] . Additionally, under such O 2 -limited conditions, chemolithoautotrophic processes that consume DIC are dominated by bacterial sulfur-driven autotrophic denitrification (SDAD) and anaerobic ammonium oxidation (Anammox), although oxygen-dependent nitrifying microorganisms (i.e., ammonium- and nitrite-oxidizers) also operate, but at lower rates [13] , [14] . In consequence, heterotrophic and chemoautotrophic processes associated with AMZs influence marine carbon dynamics and the cycling of key elements for marine productivity, but also the carbonate chemistry (pH, DIC, and p CO 2 ). The latter has been scarcely studied in these regions. For instance, heterotrophic activity reduces the efficiency of the biological carbon pump by consuming organic matter and releasing CO 2 , whereas chemoautotrophic processes can increase the efficiency of this pumping by fixing additional CO 2 and generating new organic carbon in intermediate waters [12] , [15] . Recent work has shown that the nitrite-rich AMZ in the ETSP off northern Chile is an extreme end-member within the spectrum of AMZ ecosystems, where O 2 is mostly absent, except during sporadic intrusions [10] . Gene surveys in this region have shown that significant fractions of picoplankton in AMZ waters are chemoautotrophs associated with the cycling of sulfur and nitrogen, such as SDAD and anammox [16] , [17] . Furthermore, recent studies using isotope-mixing models in other AMZs also suggest that dark carbon fixation could contribute significantly to sinking carbon fluxes [18] . However, the influence of these chemoautotrophic processes on DIC and p CO 2 levels in AMZ waters remains poorly understood. Since the biomass from chemoautotrophs inhabiting OMZs and AMZs is characterized by low δ 13 C signatures, which is modulated by both the uptake of remineralised and 13 C-depleted CO 2 [19] , and the use of carbon fixation pathways such as the acetyl coenzyme A [20] , exported organic matter from these regions should preserve this isotopically depleted signature. In view of the projected increases in both the extension and intensity of oxygen-deficient zones [7] , [8] , it remains crucial to improve our understanding about the natural variability in the carbonate chemistry system of AMZs to better predict future changes. Models suggest that a doubling of surface water p CO 2 could lead to a doubling or more of p CO 2 in OMZ/AMZ waters [21] , mostly due to the reduction of seawater´s buffer capacity by the acidic components of the normal Redfield cycle [22] . However, these projections ignore the impact of microbially driven processes linked to sulfur and/or nitrogen on biogeochemical cycles, including carbon cycling. Moreover, modeling studies based on the oceanic uptake of anthropogenic CO 2 indicate that surface waters in eastern boundary systems, such as the Humboldt Current, are likely to become more corrosive to CaCO 3 [23] . Nevertheless, the extent to which O 2 concentrations, the sulfur and nitrogen cycles, and the carbonate system are linked in AMZs remains poorly understood [12] , [15] . Here, by using a suite of physical (i.e. temperature, salinity) and chemical parameters (i.e., oxygen, inorganic nutrients, pH, total alkalinity, carbon pool concentration, and their stable isotopic composition), we hypothesize that the unique microbial communities inhabiting the AMZ ecosystem of the ETSP off northern Chile [10] , [17] constitute an important modulator of the carbonate chemistry variability in this region. These results are then incorporated into a simple carbon isotope box model to determine potential sources of organic matter and calculate the contribution of microbial autotrophic production in AMZ waters to organic carbon export to the mesopelagic region. Physical oceanographic conditions During the second half of November 2015 (austral spring; early upwelling season), coastal upwelling started its seasonal intensification, as reflected in an upwelling index of ~2000 kg m −1 s −1 off the coast of Iquique (Fig. 1c ). Sea surface temperature was ~21–22 °C, with a narrow upwelling signal < 19 °C close to the coast (Fig. 1b ). During early February 2018 (austral summer; upwelling peak) the upwelling index was ~33% stronger (3000 kg m −1 s −1 , Fig. 1e ), whereas sea surface temperatures were as low as 17 °C prevailed along the coast of northern Chile, including our coastal stations T1 and T2. These intense upwelling conditions were reflected in high surface chlorophyll a concentrations of about 20 mg m −3 within 50 km from the coastline, compared to lower concentrations of 5 mg m −3 in 2015 (Supplementary Fig. 1a , b ). Another difference between the 2015 and 2018 cruises was the hydrographic properties of the upper thermocline. Unlike 2015, the water column in 2018 was characterized by the intrusion of well ventilated, low salinity water subducted off central Chile (Supplementary Fig. 1c ) [24] . This water mass has a mean temperature of 12 °C and intrudes the upper pycnocline debilitating the AMZ, feeding the upwelling process during 2018. Anomalies of sea surface temperature for November and December 2015 did not indicate that the El Niño 2015/16 had yet arrived at the study area. Fig. 1: Sampling stations and oceanographic conditions during the expeditions. a Study area, including six sampling stations (T1–T6), and a longitudinal section from 20° down to 29.5°S, including six sampling stations (L1–L6). b 25 November–2 December 2015 composite of MODIS-Aqua SST for LowPhox I; units are in °C; persisting clouds appear in white. c Upwelling Indices for the oceanic region offshore Iquique for November 2015; black: 6-h intervals and red daily averages; units are in kg m −1 s −1 . d 2–9 February 2018 composite of MODIS-Agua SST for LowPhox II; units are in °C; persisting clouds appear in white. e Upwelling index for the oceanic region offshore Iquique from 1 January to 12 February 2018; the black lines are 6-h intervals and red dots correspond to daily averages; units are in kg m −1 s −1 . Full size image Carbon chemistry and C:N:P stoichiometry in the AMZ During 2015, oxygen-deficient conditions (<0.02 μmol kg −1 ) were observed between steep upper (~80–100 m) and lower (~400–450 m) oxyclines along the coast off northern Chile (20.0°–29.5 °S), as well as perpendicular to the coast across a neritic-pelagic transect off Iquique (20 °S; Fig. 2a ). A nitrite maximum (NO 2 − > 5 μmol kg −1 and up to 7.5 μmol kg −1 ), characteristic of anoxic conditions, was detected in the core of the AMZ between 200 and 300 m depth along the coast from ca. 20 °S to 26 °S (Station L1–L4, Fig. 1b ), as well as offshore from stations T4 to T6 (Fig. 2b ). Below the AMZ core, O 2 concentrations increased from under detection limit up to 80 μmol kg −1 (Fig. 2a ). Deficient O 2 waters were also characterized by low pH (~7.5–7.6) and high p CO 2 (~1200–1600 μatm) (Fig. 2d–f ) compared to surface oxygenated waters (pH 7.8–8.1 and p CO 2 400–700 μatm). In the AMZ core, the DIC and p CO 2 were lower, whereas pH was comparatively higher in the AMZ core around the NO 2 − maximum, compared to surrounding anoxic waters (e.g. see Stn L6, Fig. 2d, e ). Fig. 2: Spatial variability in oxygen, nitrate, and carbonate chemistry during 2015. Vertical sections of ( a ) dissolved oxygen (μmol kg −1 ), ( b ) nitrite (μmol kg −1 ), ( c ) total alkalinity (μmol kg −1 ), ( d ) pH T , ( e ), dissolved inorganic carbon (μmol kg −1 ), and p CO 2 (μatm) during the research cruise in 2015. The sections included both a cross-shelf section at 20°S (1–6), and a latitudinal section along the coast (L1–L6). The black dots represent sample locations. Full size image A comparative analysis of seawater chemistry between 2015 and 2018 in the cross-shelf transect off Iquique (20 °S; Stations T1–T6), evidenced highly contrasting conditions (Fig. 3 ). Whereas in 2015 the AMZ core (ca. 7.5 μmol NO 2 − kg −1 ) was deeper and located farther offshore, in 2018 the NO 2 − maximum (<6.5 μmol kg −1 ) was slightly shallower and closer to the coast around Stn T3, whereas the slope of both O 2 and NO 2 − isolines suggest the shoaling of low-oxygen waters over the continental shelf in 2018 (Fig. 3a–b, c–d ). High DIC concentrations were observed in subsurface waters during 2015 (>2250 μmol kg −1 ; Fig. 3e ), whereas in 2018 high DIC values were restricted to the continental shelf at Stn 1 (Fig. 3f ). The relationship between DIC and PO 4 3− concentration was relatively similar between both years as evidenced by similar slopes (Fig. 4a ). However, during 2015, some regions of the oxygen-depleted waters showed low inorganic N content (i.e., NO 3 − + NO 2 − , ~20 μmol kg −1 ) and a high N deficiency (N*; −10 to −20 μmol kg −1 ), associated with relatively lower DIC concentration (2160–2210 μmol kg −1 ) (Fig. 4b, c ). As we discuss in more detail below, high N* (>−10 µmol kg −1 ) associated with increasing DIC (~2250 µmol kg −1 ) in low-O 2 waters (filled blue dots in Fig. 4 ) appears to be related to denitrification; on the other hand, high N* values at lower DIC concentration (<2210 µmol kg −1 ) in suboxic/anoxic conditions could be associated with both SDAD and anammox processes (Fig. 4b, c ). In fact, a decrease in DIC of up to 30 μmol in the AMZ core suggests the prevalence of dark carbon fixation over heterotrophic denitrification in the DIC pool of some stations sampled during 2015 (Fig. 4b ). Moreover, since both SDAD and anammox consume H + , the high A T (2310 µmol kg −1 ), which is likely related to the consumption of nitrate and nitrite, results in the more elevated pH (~7.9) observed in oxygen-depleted waters (Stn 5) (Fig. 4d, e ). Conversely, in 2018, we observed decreasing inorganic N and high N*, but with lower DIC concentrations and high A T in comparison to 2015 (filled red dots in Fig. 4b–d ). Higher DIC concentration in the AMZ during 2015 resulted in lower pH T compared to 2018 (7.5–7.6 vs. 7.8–7.9, respectively; Fig. 4e ). Indeed, the concentration of aqueous CO 2 (CO 2-aq ; Supplementary Fig. 2a ) in the AMZ core (i.e., NO 2 − maximum) was significantly higher in 2015 (~50, and up to ~60 μmol kg −1 ) than in 2018 (~15, and up to 45 μmol kg −1 ). The relationship between O 2 and CO 2-aq in 2015 showed a large range of CO 2-aq (25–60 μmol kg −1 ) for waters with <5 μmol O 2 kg −1 , and CO 2-aq values up to 10–15 μmol kg −1 at the NO 2 − maximum (5–7.5 μmol kg −1 ; Supplementary Fig. 2a ). Fig. 3: Comparative conditions in 2015 vs. 2018 in a cross-shelf section off Iquique (20 °S). Vertical cross-shelf sections of oxygen, nitrite, dissolved inorganic carbon (DIC) and particulate organic carbon (POC) pools and their 13 C isotopic values during research cruises in 2015 and 2018. ( a , b ) Dissolved oxygen (μmol kg −1 ), ( c , d ) nitrite (μmol kg −1 ), ( e , f ) dissolved inorganic carbon (μmol kg −1 ), ( g , h ) δ 13 C DIC (‰), ( i , j ) particulate organic carbon (μmol kg −1 ), and ( k , l ) δ 13 C POC (‰). The black dots represent sample locations. Gray box represents area with non-collected data. Full size image Fig. 4: Relationship between dissolved inorganic carbon (DIC) versus nutrients and other carbonate chemistry parameters. ( a ) PO 4 3− , ( b ) inorganic nitrogen (NO 2 − + NO 3 − ), ( c ) N*, ( d ) total pH (pH T ), and ( e ) total alkalinity (A T ), within the range from surface to 1000 m water depth during 2015 and 2018 expeditions. Filled symbols correspond to data points associated with O 2 concentrations < 20 μmol kg −1 . The correlations observed in low oxygen waters (filled points) for DIC versus nitrogen at 2015 is given and indicated by the dark blue line ( b ). Labels in ( b ) were included to emphasize the processes highlighted in the stoichiometric analysis (e.g. Annamox, sulfur-driven autotrophic denitrification (SDAD), and denitrification). Full size image During both years, suspended POC concentrations decreased by 15–20 μmol kg −1 over the upper 100 m of the water column and remained low (ca. 5 μmol kg −1 ) through the OMZ (Fig. 3i, j ). Contrasting concentration profiles between both years were also observed. In 2015, surface POC was <18 μmol kg −1 , whereas in 2018 it reached values up to 32 μmol kg −1 (Fig. 3i, j ). These trends were also reflected in chlorophyll-a concentrations, which exhibited lower (< 5 μg L −1 ) values in the coastal area (Stn T1 and T2) in 2015, whereas higher (up to 11.8 μg L −1 ) and more spatially distributed concentrations (from Stn T1 to T3) were observed in surface waters during 2018 (Supplementary Fig. 3 ). Isotopic signature of DIC and POC The stable isotope composition of DIC and POC from the cross-shelf transect near Iquique (20 °S; Stations T1–6) showed contrasting conditions between both sampling periods (Fig. 3 ). In 2015, isotopically depleted δ 13 C DIC values (0.0 to −0.5 ‰) and high DIC concentrations (>2250 μmol kg −1 ) were observed within the AMZ, but particularly in the upper core region (e.g., Stn T3, 100–200 m; Fig. 3g ). Isotopically depleted δ 13 C DIC values were also observed at depth in 2018, but mostly associated with the coastal area (Stns T1 and T3), and between 100 and 400 m depth (Fig. 3h ) along with the highest concentration of NO 2 − (Fig. 3d ). During 2018, we observed even more isotopically depleted δ 13 C DIC values (−0.6 to −0.8 ‰) and slightly lower, yet still high, DIC concentrations (<2200 μmol kg −1 ) compared to 2015 (Fig. 3g, h ). The observed relationship between DIC concentration and δ 13 C DIC (Supplementary Fig. 2b ) suggests that δ 13 C DIC is primarily governed by biological uptake in oxygenated waters (>20 μmol kg −1 ) and by microbial respiration in low O 2 waters (<20 μmol kg −1 ), with the most depleted δ 13 C values associated with low oxygen and high p CO 2 waters. The difference in δ 13 C POC values between both years was larger than in δ 13 C DIC . The δδ 13 C POC in the upper 50 m ranged between −23‰ and −27‰ in 2015 and from −18.5‰ to −20.5 ‰ in 2018, with the most positive δ 13 C POC values in the euphotic zone (Fig. 3k, l ). These values are within the reported range of 13 C fractionation due to photosynthetic carbon fixation [25] , [26] . However, within the AMZ core, and lower deep oxycline, we observed contrasting differences in δδ 13 C POC values between both years. During 2015, δ 13 C POC values were as low as −32‰ (Fig. 3k ), particularly at 300 m depth at Stn 2, and down to 400 m at Stn 6. Notably, even more isotopically depleted δ 13 C POC values were detected in oxic deep waters below the AMZ and down to 1000 m (Stn 6; Fig. 3k ). On the other side, during 2018, δ 13 C POC values within the AMZ core and deeper waters were more isotopically enriched and ranged from −23 to −28 ‰ (Fig. 3l ). The estimated values of δ 13 C CO2 , as well as the respective isotopic fractionation ( ε ) against 13 C between CO 2 and POC, and DIC and POC, show contrasting conditions both through the water column of each year and between both years, especially below the lower oxycline (down to 400 m depth; Supplementary Fig. 4 ). In 2015, from the lower deep oxycline down to 1000 m depth, ε values varied ~21–23‰ and ~32–33‰ for CO 2 -POC and DIC-POC, respectively (Supplementary Fig. 4c, e ). In 2018, ε values were ~17‰ and <24‰ for CO 2 -POC and DIC-POC over almost the entire water column, respectively (Supplementary Fig. 4d, f ). Calcium carbonate saturation state We observed distinct conditions for calcium carbonate saturation state (Ω) between both expeditions. During 2015, waters below 100 m were corrosive for aragonite, as depicted by Ω arag < 1.0 (Fig. 5a ) and low pH values < 7.8 (Fig. 2d ). However, the calcite saturation horizon (Ω calc < 1.0) was not observed in the upper 1000 m of the water column during both years (Fig. 5c, d ). In 2015, both Ω arag and Ω calc were low at the lower deep oxycline between 350 and 450 m depth (Fig. 5a, c ). Contrarily, both aragonite and calcite-undersaturated conditions were not observed in the water column in 2018, with a shoaling towards the coast (at 100 m depth in Stn 1), while Ω arag values < 1.0 were observed in bottom waters (Fig. 5b ). Fig. 5: Calcium carbonate saturation state during both research cruises. Vertical cross-shelf sections of ( a , b ) aragonite saturation state (Ω arag ) and ( c , d ) calcite saturation state (Ω cal ) during research cruises in 2015 and 2018. The dotted red line for Ω values represents the isopleths of 1; below such value is considered CaCO 3 undersaturation. The black dots represent sample locations. Gray box represents an area with non-collected data. Full size image Model We used a simple carbon isotope mass balance model to determine the potential sources of microbially produced organic matter within AMZ waters, and to estimate how much of this carbon is exported to deeper waters in this region. The results of our carbon isotope model demonstrate that the potential contribution of microbial production to carbon export varies greatly (~7–35%), which relies on a net fractionation factor (ε Famz ) of carbon fixation via autotrophic production in the AMZ, and the relative proportion of carbon fixed as HCO 3 vs CO 2 (Fig. 6 ). 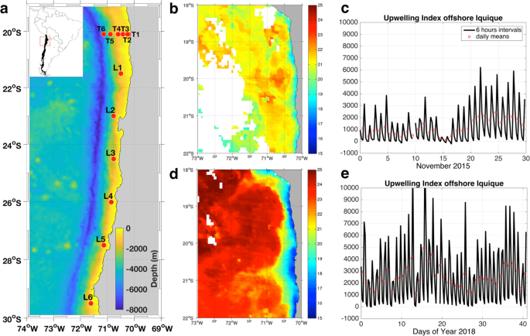Fig. 1: Sampling stations and oceanographic conditions during the expeditions. aStudy area, including six sampling stations (T1–T6), and a longitudinal section from 20° down to 29.5°S, including six sampling stations (L1–L6).b25 November–2 December 2015 composite of MODIS-Aqua SST for LowPhox I; units are in °C; persisting clouds appear in white.cUpwelling Indices for the oceanic region offshore Iquique for November 2015; black: 6-h intervals and red daily averages; units are in kg m−1s−1.d2–9 February 2018 composite of MODIS-Agua SST for LowPhox II; units are in °C; persisting clouds appear in white.eUpwelling index for the oceanic region offshore Iquique from 1 January to 12 February 2018; the black lines are 6-h intervals and red dots correspond to daily averages; units are in kg m−1s−1. 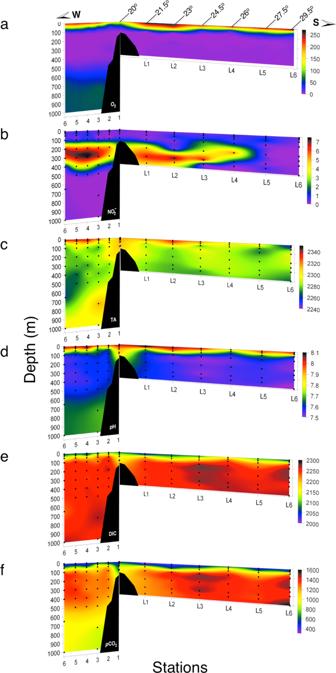Fig. 2: Spatial variability in oxygen, nitrate, and carbonate chemistry during 2015. Vertical sections of (a) dissolved oxygen (μmol kg−1), (b) nitrite (μmol kg−1), (c) total alkalinity (μmol kg−1), (d) pHT, (e), dissolved inorganic carbon (μmol kg−1), andpCO2(μatm) during the research cruise in 2015. The sections included both a cross-shelf section at 20°S (1–6), and a latitudinal section along the coast (L1–L6). The black dots represent sample locations. By incorporating depth integrated carbon fixation rates of each prominent autotrophic metabolism in the AMZ (see Table 1 ), we applied a weighted average to estimate the net fractionation associated with AMZ autotrophy (ε Famz : see Table 2 ) under two contrasting scenarios. Since AMZ systems are temporally variable, the two scenarios reflect the different possible ranges of metabolic rates between distinct seasonal conditions in 2015 and 2018 (i.e. high SDAD vs low SDAD, respectively). The model results demonstrate a significant difference in the microbial contribution to organic carbon export below the AMZ between years, ranging from ~2-17% greater in 2015 than 2018 (Fig. 6 ). This marked difference in the potential microbial contribution to POC below the AMZ (as much as double in 2015 than 2018) appears to be largely driven by the systematically heavier δ 13 C POC (~5‰ across all depths) in 2018, likely a result of an increased phytoplanktonic contribution to the organic carbon pool. Fig. 6: Summary results of carbon isotope model under range of inorganic carbon conditions and Low/High SDAD Scenarios. ε Famz indicates the net fractionation factor based on a weighted average of each autotrophic metabolism expected to be active in the AMZ. Shaded areas denote error estimates in ε Famz derived from the mean fractionation factors of individual autotrophic metabolisms. Full size image Table 1 Depth integrated carbon fixation rates (µmol C m −2 d −1 ) present in the AMZ of northern Chile incorporated in our isotope mass balance model for weighting of the ε Famz variable. Full size table Table 2 Variables incorporated into the calculation of f onet across all inorganic carbon conditions and under two scenarios of relative carbon fixation rates. Full size table The remineralization rates in the euphotic zone and AMZ have a significant impact on the calculations of microbial contribution; as values approach complete recycling of AMZ-produced carbon (AMZ Remineralization = 100%), the contribution of microbial production expectedly approaches 0% (see Eq. 3 ). Remineralization in the euphotic zone is kept at 95% in all conditions to reflect realistic degradation rates of surface-derived organic matter in this region at 300 m [27] , meaning that ~5% of what is produced in the surface is exported to the AMZ (see Table 2 ). The fixation of HCO 3 − vs CO 2 in the euphotic zone has no effect between model runs; the 13 δC POC in the surface remains the same as the ε Fez is adjusted to remain consistent with the measured isotopic composition of the organic carbon pools. However, the model also demonstrates that the form of inorganic carbon utilized in the AMZ has a significant impact on the isotopic composition of POC in the AMZ, and thus the estimated total microbial contribution (Fig. 6 ). By incorporating relative contributions determined from the total range of metabolic rates reported in the literature for each autotrophic process present in the ETSP AMZ, we estimate the microbial contribution to organic carbon export to range between ~7 and 18% in the 2018 cruise, and between ~9 to 35% in the 2015 cruise (Table 2 and Fig. 6 ). Geochemical and stable isotope data from two expeditions to the AMZ off northern Chile with contrasting oceanographic regimes highlight the biogeochemical variability of this environment. The interaction of local processes, such as the strength and spatial variation of upwelling conditions [28] , and its interconnection with regional processes, such as the intensity and displacement of mesoscale eddies [29] , in addition to the advection of tropical waters, determine surface productivity and the variability of the zonal and vertical boundaries of the AMZ core. The latter can in turn influence carbon cycling and export in this region – i.e., the source and fate of different carbon pools through the water column. Previous studies in the area have shown the accumulation of nitrite (>0.5 μmol kg −1 ) [13] in oxygen-free waters [30] between 200 and 300 m depth along the coast (ca. 20–26 °S). Anoxia is maintained by both the remineralization of organic matter produced in surface waters and the low ventilation due to strong stratification [31] , [32] . Anoxic waters were characterized by low pH and high p CO 2 conditions (pH < 7.5 and p CO 2 > 1200 µatm), which places the AMZ of the ETSP as one of the most oxygen-deficient and acidic systems worldwide [32] , [33] , [34] , [35] . Carbonate chemistry in the AMZ is also highly temporal and spatially variable, as reflected by the contrasting levels of DIC concentration and pH between austral spring 2015 and summer 2018. Our results evidence that the ETSP AMZ off the coast of northern Chile embodies one of the shallowest (~100–400 m depth), low pH, high p CO 2 AMZ systems in the world [5] , similar to what has been observed off the Peruvian coast [29] . Indeed, the aragonite saturation depth can be as shallow as 100 m depth, as observed during austral spring in 2015. The position of the AMZ core is also dynamic, with an AMZ core farther offshore during 2015 and more restricted to the continental shelf in 2018. Notably, during 2015 we observed a decrease in DIC and aqueous CO 2 (CO 2-aq ) concentrations down to ~30 µmol kg −1 in the AMZ core relative to adjacent, similarly oxygen-depleted waters (Supplementary Fig. 2A ). In the same study area, Paulmier et al. [12] observed a similar carbon deficit associated with the OMZ, which they related to oxygen loss due to thermal mechanisms during OMZ water formation in the equatorial region, since a decrease in DIC is expected in warm regions due to a lowering of gas solubility. Indeed, when we analyze p CO 2 data collected in the ETSP between 7 and 15 °S [29] shows a steady reduction in p CO 2 as the Equatorial Subsurface Waters (ESSW) move southward along the Peruvian coast. Here, we explore the hypothesis that microbial processes involved in sulfur and nitrogen cycling can exert an additional partial control for such DIC deficit. For instance, the generally increased DIC concentrations in high-N* and low-O 2 waters suggests active organic matter respiration via nitrate reducers, with the canonical denitrification pathway responsible for part of the N* registered in both years (>–20 µmol kg −1 ), which was remarkably high during 2018 (up to –40 µmol kg −1 ). Thus, while organic matter remineralization is expected to reduce alkalinity due to proton production, the observed high A T in both years could be explained by a net nitrate input from an external source feeding nitrate reducers and denitrifiers [36] , as expected to occur particularly during the upwelling-active period registered in 2018. Inversely, the low DIC concentrations in the O 2 -depleted and N-deficient waters observed in some stations (Stns 5-6) during 2015 could be associated with dark carbon fixation. The δ 13 C DIC and δ 13 C POC data suggest that chemosynthetic processes, which could reduce p CO 2 in the AMZ [36] , [37] , were likely more dominant during 2015. It is well known that AMZs host an active and diverse autotrophic and heterotrophic microbial community [10] , [13] . Indeed, the unusually depleted δ 13 C POC values, along with the ε values for CO 2 /DIC and POC observed in the AMZ core in 2015, reinforce the idea that inorganic carbon fixation processes such as SDAD and anammox [20] , previously reported to be active in oxygen-deficient regions [38] , [39] , might significantly influence the carbonate chemistry of AMZs. However, the low carbon fixation rates estimated through anammox [15] ( ∼ 0.0004 µmol C L −1 d −1 ; based on a C:N = 0.066/1) compared to SDAD (from 0.3 up to 20 µmol C L −1 d −1 in the ETSP off Peru and Chile; Supplementary Table 1 ), support the idea that SDAD, with a higher carbon isotopic fractionation factor (mean of −24.8‰ [40] ) than anammox (mean of −18.2‰ [20] ), could be the dominant chemolithoautotrophic process driving carbon fixation in the AMZ. Although some studies suggest that SDAD can only be important in coastal AMZ waters [41] , sulfide oxidation rates calculated for the same study area (i.e. although with sulfide concentrations higher than in situ conditions) were high (i.e. relative to anammox and denitrification rates), and strongly coupled to nitrate reduction [13] . High sulfide oxidation activity has also been linked to metagenome analysis in our study area, which indicates the occurrence of enriched sequences matching the genomes of sulfur-oxidizing endosymbionts lineages (i.e. like Candidatus Ruthia magnifica , Candidatus Vesicomyosocius okutanii , and SUP05 pelagic linage), especially during spring/summer conditions [10] , [13] , [16] , such as in our 2015 expedition (i.e. austral spring). It has been suggested that sulfide oxidation is mainly sustained by sulfate reduction; however, the undetectable sulfide accumulation in OMZ/AMZ waters seems to be associated with its immediate oxidation back to sulfate, or to different sulfur intermediate compounds [42] , as part of what has been described as a cryptic sulfur cycle [13] . Furthermore, offshore SDAD activity could also be supported by eddy-driven zonal advection (i.e. a mesoscale process particularly active for northern Chile [43] ) of SUP05 species and hydrogen sulfide that is frequently accumulated in OMZ shelf waters [39] , [44] . Actually, mesoscale eddies in this region can persist for weeks or months [45] . Moreover, Stn T5 is only ~75–80 km offshore. Therefore, a conservative estimate of sulfide oxidation using the ranges reported by both Canfield et al. [13] and Callbeck et al. [39] off northern Chile and Peru, respectively, as well as mean anammox rates for the same area [46] , [47] , [48] , [49] , [50] , suggests that dark carbon fixation could remove from 0.12 up to 0.63 µmol C L −1 day −1 during the southward travel of the ESSW. A study in the ETNP OMZ off Mexico [51] also reported high DIC assimilation at the OMZ core (6.4 µmol C L −1 d −1 ) in association with depleted δ 13 C POC values (−30.3‰), which they assigned to anammox activity based on molecular biomarkers analyses. However, Cavan et al. [52] already suggested that anammox is unlikely to be solely responsible for dark carbon fixation in OMZ waters offshore. As stated above, the low anammox rates reported for our study area suggest that this metabolism plays a rather neglectable role in the DIC deficit in the core AMZ, despite the fact that enough NH 4 + , the apparent limiting substrate, is produced in the ETSP off northern Chile (Supplementary Table 2 ). Our results provide a robust biologically mediated mechanism for the observed DIC variability found in AMZs (deficit or accumulation), although we cannot rule out additional processes (biological/physical). Aerobic NH 4 + oxidizers, considered to be the main chemoautotrophs in the ocean [53] , have an ε similar to anammox (mean of 19.3‰ [54] ), and they can support up to 50% of the total dark carbon fixation in the upper oxycline of the ETSP AMZ [55] . However, the contribution of this process to carbon cycling within the AMZ is likely neglectable, as its activity [55] , [56] , [57] and the abundance and expression of genes that regulate this pathway [10] , [16] , [56] decrease with depth in the AMZ. For instance, NH 4 + oxidation rates drop three orders of magnitude in experiments using water from the oceanic AMZ oxycline (250 μmol O 2 L −1 ; 800 nmol N L −1 d −1 ) [55] , the upper AMZ (<5 μmol O 2 L −1 ; 150 nmol N L −1 d −1 ), and the AMZ core (6 nmol O 2 L −1 ; 4 nmol N L −1 d −1 ) [57] . At depressed rates, NH 4 + oxidizers fix 0.5 nmol C L −1 d −1 (based on a C:N ratio = 1.0:8.3) [58] , which is three orders of magnitude lower than the mean C fixation estimated for SDAD in the AMZ (see Supplementary Table 2 ). Nevertheless, since part of the particulate material settled to the AMZ could have the δ 13 C imprint from NH 4 + oxidizers at the oxycline and/or at the upper OMZ boundary, its potential contribution to the organic carbon pool in the AMZ should be considered. Increased A T (>2300 µmol kg −1 ) and high DIC concentrations (>2200 µmol kg −1 in some samples) in O 2 -depleted and N-deficient waters suggest a predominance of heterotrophic denitrification over autotrophic processes during 2018. Furthermore, the ε values between CO 2 and POC, as well as between DIC and POC, were significantly lower than in 2015 over almost the entire water column (17‰ and 24‰, respectively). Therefore, and considering the higher phytoplankton and POC biomass in surface waters during 2018, our results suggest that most (or at least a significant fraction) of the organic carbon exported to the AMZ and below derives from recently settled photosynthetically-fixed carbon in surface waters [25] , [26] , [59] . This fresh organic material might have stimulated the heterotrophic community, particularly the fast-growing denitrifiers [49] , [60] (i.e. relative to the slow growing anammox bacteria [61] ). This argument is also confirmed from previous studies in the same region [49] , [60] , where the highest denitrification rates were found associated with areas with high chlorophyll levels in the euphotic zone. In general, N cycling in the AMZ is tightly coupled to the organic matter produced and exported from the surface [60] . The dominant microbial functional types found in the AMZ core of this region have the potential for sulfur/ammonium oxidation, nitrate/nitrite reduction, and especially inorganic carbon fixation (C1 carbon fixation) [10] , with denitrification, anammox, and sulfur oxidation pathways as the dominant processes in the core of the AMZ [10] , [13] . SUP05 and SAR324 are well-known bacterial clades with the metabolic flexibility to perform bicarbonate (DIC) uptake [13] , [62] as well as methane oxidation [63] , and they are common in this oxygen-limited system [10] . 15 N-tracer approaches have confirmed active N-loss through denitrification and anammox in this region [48] , [50] , [64] , although both processes exhibit high spatiotemporal variability in this and other AMZ systems [65] , [66] , [67] . In general, anammox, which is particularly predominant in the ETSP, is highly active just below the upper AMZ boundary, and declines exponentially with depth [48] , [49] . However, no depth dependence has been discerned for denitrification [49] . On the other hand, beyond oxygen limitation [47] , [68] , [69] , the input of electron donors exerts a main control of N-removal processes, i.e., organic matter quality and lability [60] , [70] , NH 4 + availability from organic matter remineralization [46] , [48] , [56] , [60] , and sulfide readiness [13] , [38] . Thus, the observed variability in the dominance of different microbial processes between 2015 and 2018 is likely associated with the seasonal oceanographic dynamic reported for AMZ waters in this region [28] , [71] . Our 2015 sampling occurred during austral spring conditions and under a moderated upwelling regime with a narrow upwelling signal at the coast, whilst the 2018 sampling occurred during an intense summer upwelling event with high productivity in surface waters (20 mg Chl-a m −3 ). The export of organic matter from dark carbon fixation processes occurring in AMZ waters to deeper layers of the ocean may contribute to the depleted δ 13 C POC signatures found in waters below the AMZ in 2015. A recent organic geochemical study in the AMZ off northern Chile [72] reported that a biomarker specific of anammox bacteria [73] was not only abundant in the suspended organic matter within AMZ waters, but also in oxygenated waters below, possibly indicating the occurrence of exported biomass from the AMZ, and/or active anammox bacteria in anoxic microniches within sinking particles. However, the lack of robust biomarkers for SDAD makes a quantitative comparison of the relative contribution of anammox vs. SDAD to POC using biomarkers in AMZ regions still difficult. Our carbon isotope-mixing model investigated the potential contribution of microbial autotrophs in AMZ waters based on the net isotopic fractionation factor (ε Famz ) during carbon fixation. The model includes contributions from low light-adapted cyanobacteria, anammox bacteria, nitrifying archaea/bacteria, and sulfide-oxidizing bacteria during the two cruises. The carbon chemistry and C:N stoichiometries from the 2015 and 2018 cruises suggest a dynamic shift, in terms of carbon fixation, from a SDAD dominated AMZ to a largely photoautotrophic/nitrifying system. Thus, we applied the carbon isotope model under two distinct scenarios, a relatively high SDAD scenario to reflect the conditions in the 2015 cruise, and a low SDAD scenario in 2018 (Table 2 ). In order to constrain the potential range of total microbial contribution to carbon export, we compared depth-integrated metabolic rates of chemoautotrophy in the AMZ under these two generalized scenarios (Table 1 ). The model results indicate that the total microbial contribution from AMZ waters to carbon export likely ranged between ~7 and 18% in the 2018 cruise, and between ~9 and 35% in the 2015 cruise (Fig. 6 ). 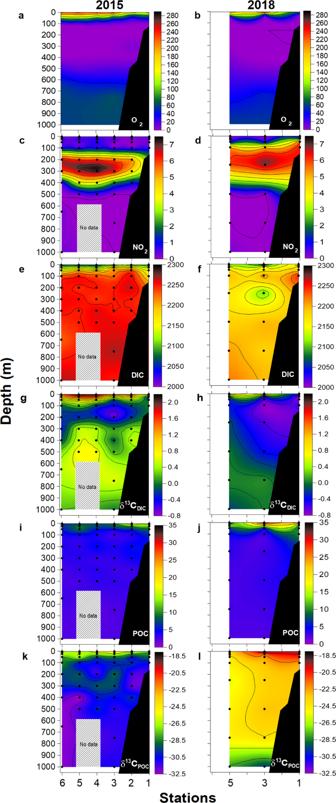Fig. 3: Comparative conditions in 2015 vs. 2018 in a cross-shelf section off Iquique (20 °S). Vertical cross-shelf sections of oxygen, nitrite, dissolved inorganic carbon (DIC) and particulate organic carbon (POC) pools and their13C isotopic values during research cruises in 2015 and 2018. (a,b) Dissolved oxygen (μmol kg−1), (c,d) nitrite (μmol kg−1), (e,f) dissolved inorganic carbon (μmol kg−1), (g,h) δ13CDIC(‰), (i,j) particulate organic carbon (μmol kg−1), and (k,l) δ13CPOC(‰). The black dots represent sample locations. Gray box represents area with non-collected data. Our estimates provide quantitative evidence for a significant and novel secondary source of organic carbon exported to the mesopelagic region from oxygen-deficient waters that have been generally overlooked. Recently, using intact polar lipids in size-fractionated POM, Cantarero et al. [74] suggested that the standing stock of microbial biomass in AMZ waters of this system might be larger than that of the oxic photic zone, thus supporting the notion that dark carbon fixation might contribute to carbon export to the deeper ocean. Indeed, Lengger et al. [75] demonstrated that organic carbon produced through chemoautotrophic carbon fixation could constitute a substantial proportion (17%) of the organic matter exported from the Arabian Sea OMZ to underlying surface sediments. It has been suggested that similar to episodes of transient warming in earth history, modern and future ocean warming could impact the oceanic biological pump, largely via increasing surface ocean temperature [76] , a reduction in the remineralization depth [77] , [78] , and therefore reduced CO 2 storage [76] . Our results highlight the potential implications of enhanced microbial processes in AMZ waters [77] as a source of isotopically depleted organic carbon that has not been considered when estimating changes in carbonate chemistry and carbon cycling in projections of AMZ expansion. Moreover, dark carbon fixation by microorganisms involved in nitrogen, carbon, and sulfur cycling could also influence, through dark carbon fixation, the carbonate chemistry conditions (pH, A T , and p CO 2 ) for temporary or permanent AMZ inhabitants [79] . Thus, the recent evidence for decreasing pH due to reduced ventilation in the deep ocean [80] deserves revision in some oceanic regions, since such conclusions do not consider the role of microbially mediated biogeochemical processes associated with sulfur and nitrogen cycles, which can modify the carbonate chemistry in AMZ waters at depth. In consequence, there is a need for new biogeochemical models that take into account sulfur/nitrogen-driven microbial processes occurring in AMZs under future scenarios of ocean change. Field sampling and hydrographic profiles Samples were collected during two expeditions to the ETSP off northern Chile during late November 2015 (LowpHOX 1) and February 2018 (LowpHOX 2) onboard the R/V Cabo de Hornos . The sampling design during 2015 considered an inshore-offshore transect off Iquique (20 °S) with six sampling stations (T1–T6), and a longitudinal transect with six sampling stations (L1–L6) from 20° down to 29.5 °S (Fig. 1 ). During 2018 we studied three sampling stations along the inshore-offshore transect (T1, T3, and T5). Hydrographic profiles were recorded during both cruises using the same SeaBird SBE-911+ CTD system equipped with two temperature and conductivity sensors, a SBE 43 oxygen sensor and fluorometer, and 24 10-L General Oceanic Niskin Bottles. Temperature and conductivity sensors were pre-cruise calibrated. The raw data were processed following the recommended procedures provided by the manufacturer and were averaged into one dbar bins. Additionally, a pump profiling system (PPS) was also used for water collection and high-resolution O 2 measurement. Upwelling index and MODIS images The Upwelling Index is based on Ekman Transport estimates provided by NOAA ERDDAP ( http://coastwatch.pfeg.noaa.gov/erddap/griddap/erdlasFnTran6.html ). The horizontal resolution of the transport estimates is 1 × 1° latitude × longitude on a 6-h interval. We chose the grid point at 20.5 °S and 70.5°W offshore Iquique. The Upwelling Indices were calculated with an algorithm published by NOAA ERDDAP on their website. The data to compute Sea Surface Temperature and Chlorophyll-a maps were obtained from the MODIS-Aqua website https://oceandata.sci.gsfc.nasa.gov/MODIS-Aqua/Mapped/8-Day/4km/ . MODIS (or Moderate Resolution Imaging Spectroradiometer) is a key instrument aboard the Terra (originally known as EOS AM-1) and Aqua (originally known as EOS PM-1) satellites. Terra’s orbit around the Earth is timed so that it passes from north to south across the equator in the morning, while Aqua passes south to north over the equator in the afternoon. Terra MODIS and Aqua MODIS screen the Earth’s surface every 1–2 days, acquiring data in 36 spectral bands, or groups of wavelengths (see MODIS Technical Specifications). The horizontal resolution of the database is 4 × 4 km and 8-day composites of cloud-free ocean are provided. Chlorophyll a, dissolved nutrients, and elemental stoichiometry Chlorophyll a concentration and dissolved inorganic N (nitrite, NO 2 − and nitrate, NO 3 − ) and phosphate (PO 4 3− ) were analyzed using standard protocols [81] , [82] . In order to calculate the deviation from the classical Redfield ratio (N:P = 16:1) (Redfield et al. 1963), we calculated the tracer N* [83] (Eq. 1 ): 
    N∗ = ([ NO_3^ - ]-16 ×[ PO_4^3 - ] + 2.9) × 0.87
 (1) where [NO 3 − ] and [PO 4 3− ] are the concentrations of nitrate and phosphate in μmol kg −1 , respectively. Positive and negative N* are an indicator of an excess or deficit of NO 3 − relative to PO 4 3− [82] , respectively, and values are typically arbitrary units rather than absolute concentrations. Carbon pools and stable isotope analyses Samples for pH T were collected in 50 mL syringes and immediately transferred to a 25 mL thermostatted cell at 25.0 ± 0.1 °C for standardization, with a pH meter Metrohm® using a glass combined double junction Ag/AgCl electrode (Metrohm model 6.0258.600), which was calibrated with 8.089 Tris buffer solution as a certified reference material (CRM, supplied by Andrew Dickson, Scripps Institution of Oceanography, San Diego, USA) at 25 °C. pH values are reported on the total scale (pH T ). Samples for total alkalinity (A T ) were poisoned with 50 µL of saturated HgCl 2 solution and stored in 500 mL borosilicate BOD bottles with ground-glass stoppers lightly coated with Apiezon L ® grease and kept in darkness and room temperature. A T was determined using the open-cell titration method [84] , by using an automated Alkalinity Tritrator Model AS-ALK2 Apollo SciTech. All samples were analyzed at 25 °C ( ± 0.1 °C) with temperature regulation using a water-bath. Analytical accuracy was controlled against a certified reference material (CRM, supplied by Andrew Dickson, Scripps Institution of Oceanography, San Diego, USA) and the A T repeatability averaged 2-3 µmol kg −1 . DIC samples were collected in 250 mL Wheaton® glass bottles and preserved with 50 μL saturated HgCl 2 solution. Immediately after opening the sample bottle, a digital syringe withdrew a small volume (0.5 ml), acidified it with 10% phosphoric acid and subsequently measured the evolved CO 2 with a LICOR 6262 non-dispersive infrared gas analyzer. 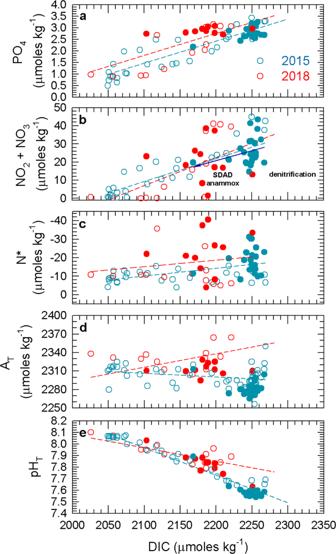Fig. 4: Relationship between dissolved inorganic carbon (DIC) versus nutrients and other carbonate chemistry parameters. (a) PO43−, (b) inorganic nitrogen (NO2−+ NO3−), (c) N*, (d) total pH (pHT), and (e) total alkalinity (AT), within the range from surface to 1000 m water depth during 2015 and 2018 expeditions. Filled symbols correspond to data points associated with O2concentrations < 20 μmol kg−1. The correlations observed in low oxygen waters (filled points) for DIC versus nitrogen at 2015 is given and indicated by the dark blue line (b). Labels in (b) were included to emphasize the processes highlighted in the stoichiometric analysis (e.g. Annamox, sulfur-driven autotrophic denitrification (SDAD), and denitrification). Certified seawater reference materials from A. Dickson were used to ensure the quality of DIC determination by preparing a calibration curve covering the range of DIC from 200–2000 μeq L −1 , with a resulting precision averaging ≈ 0.1% (range 0.05–0.5%). Temperature, salinity, A T, and DIC data were used to calculate aqueous CO 2 (CO 2 -aq), p CO 2 , and Calcite Saturation State (Ω calcite ) Analyses were performed using CO 2 SYS software for MS Excel [85] set with Mehrbach solubility constants [86] refitted by Dickson & Miller [87] . The KHSO 4 equilibrium constant determined by Dickson [88] was used for all calculations. Stable isotopic (δ 13 C) measurement of DIC was performed following a method modified version of the method by Torres et al (2015) [89] . Seawater DIC samples were collected in 250 mL Wheaton® glass bottles and preserved with 50 μL saturated HgCl 2 solution. Inside a glove bag, 1 mL water sample was transferred into pre-cleaned (10% HCl-rinsed and 540 °C/4 hrs combusted) 12 mL Exetainer® vials and then capped before sealing the vial with an ultra-high purity helium headspace. DIC samples were acidified with 50 µL 85% H 3 PO 4 via syringe injection through the septum, and allowed to equilibrate at room temperature for 12 hours. Evolved headspace p CO 2 δ 13 C DIC was then measured using a Gas Bench II and a Finnigan Delta Plus isotope ratio mass spectrometer at UC Irvine, with an analytical uncertainty of ± 0.05‰. In order to estimate the isotopic signature of CO 2 incorporated during uptake, we also estimated the δ 13 C of ambient CO 2 (aq) by using the Eq. 2 derived from Rau et al. [90] : 
    δ ^13C_CO2 = δ ^13C_DIC + 23.644-( 9701.5/T_K)
 (2) where δ 13 C DIC is the δ 13 C of ambient DIC and T K is the corresponding temperature in Kelvin scale. Seawater samples (500–1000 mL) were collected by vacuum filtration through pre-combusted (4 h at 450 °C) MFS GF/F glass fiber filters (0.7 µm nominal pore size, 25 mm diameter) for POC analyses. Prior to filtration, filters were rinsed with 10% HCl followed by deionized water to eliminate any trace of inorganic carbon. In 2015 cruise, POC concentration and δ 13 C POC were determined at the Stable Isotope Facility at the University of California Davis by using an Elementar Vario EL Cuve or Micro Cube elemental analyzer (Elementar Analysensysteme GmbH, Hanau, Germany) interfaced to a PDZ Europa 20–20 isotope ratio mass spectrometer (Sercon Ltd., Cheshire, UK). The long-term precision reported is ±0.2‰ for δ 13 C POC in this range with precision decreasing on the lower end. POC concentration and the δ 13 C POC for the 2018 cruise filtrates were measured using a Thermo Scientific Elemental Analyzer—Isotope Ratio Mass Spectrometer at the CU Boulder Earth Systems Stable Isotope Lab. Purified acetanilide, ethylenediaminetetraacetic acid, and in-house (Pugel) standards were measured for external calibration and drift corrections with a total carbon and nitrogen analytical precision between 1.1–2.2% and 0.6–2.2%, respectively, and a δ 13 C POC analytical precision between 0.09 and 0.17‰ across all analysis runs. During analysis, samples are interspersed with several replicates of at least two different laboratory standards. Model We utilized a carbon isotope mass balance model to determine potential sources of organic matter and estimate the impact of microbial dark autotrophic production to carbon export from the AMZ (Eqs. 3 , 4 and 5 ); where ez is the euphotic zone, amz the anoxic marine zone, Ф represent the mass fluxes (P-primary productivity, R-respiration), r e is the remineralization in the euphotic zone, r o the remineralization in OMZ), δ is the isotopic composition of carbon pool, ε is the fractionation factor (F-carbon fixation, R-respiration), OC is the organic carbon, and DIC the dissolved inorganic carbon concentration. The exported carbon pool in the mesopelagic region is described as a ratio of fluxes between net-AMZ and -total net primary production (i.e. euphotic zone + AMZ net primary production; Eq. 3 ). Remineralization rates are defined as the relative fluxes of respiration/production (Eq. 4 ). The contribution of productivity in the AMZ to carbon export ( f onet ) is defined in terms of: the net productivity fluxes, the isotopic fractionation factors (ε) of carbon fixation and respiration in the euphotic zone and AMZ, and the isotopic composition of the organic and inorganic carbon pools in both the euphotic zone and AMZ (Eq. 5 ). The measured δ 13 C of bulk organic matter and total dissolved inorganic carbon from both the euphotic and AMZs along the 2015 + 2018 oceanographic expeditions are fed into Eq. 3 under a range of inorganic carbon conditions and 2 different scenarios of metabolic activity. We calculated f onet assuming different proportions of HCO 3 and CO 2 utilized in carbon fixation from AMZ autotrophy expressed as a ratio (HCO 3 :CO 2 fixation) from 0 to 1. 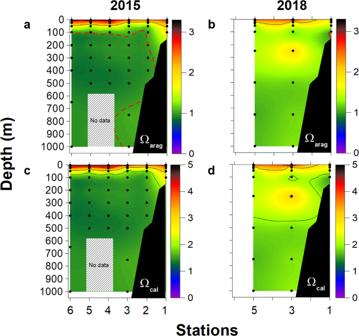Fig. 5: Calcium carbonate saturation state during both research cruises. Vertical cross-shelf sections of (a,b) aragonite saturation state (Ωarag) and (c,d) calcite saturation state (Ωcal) during research cruises in 2015 and 2018. The dotted red line for Ω values represents the isopleths of 1; below such value is considered CaCO3undersaturation. The black dots represent sample locations. Gray box represents an area with non-collected data. 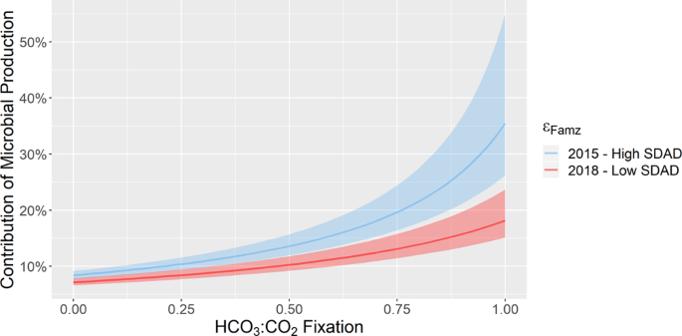Fig. 6: Summary results of carbon isotope model under range of inorganic carbon conditions and Low/High SDAD Scenarios. εFamzindicates the net fractionation factor based on a weighted average of each autotrophic metabolism expected to be active in the AMZ. Shaded areas denote error estimates in εFamzderived from the mean fractionation factors of individual autotrophic metabolisms. In addition, we calculated f onet under two scenarios (High SDAD and Low SDAD) by estimating an ε Famz value derived from a weighted average from depth integrated rates of carbon fixation from each autotrophic metabolism active in the AMZ (see Table 1 for summary of model conditions and scenarios). f_onet = Φ_amzPΦ_amzR/Φ_amzP - Φ_amzR + Φ_ezP - Φ_ezR
 (3) 
    r_e = _Rez/_Fez; r_o = _Ramz/_Famz
 (4) 
    f_onet = (r_o - 1)(δ _OCez - δ _OCamz)/(r_o - 1)δ _DICez + δ _DICamz - ϵ_Fez + r_eϵ_Rez + ϵ_Famz - r_o(δ _OCamz - ϵ_Fez + r_eϵ_Rez + ϵ_Ramz)
 (5) The autotrophic metabolisms present with significant carbon fixation rates within the AMZ in these model runs are limited to low light-adapted cyanobacteria, nitrifying bacteria/archaea, anammox bacteria, and sulfur-oxidizing bacteria. Average fractionation factors for each autotroph’s respective carbon fixation pathway [20] , [40] , [54] , [91] , [92] are incorporated into the model (Table 1 ) and expressed as a weighted average (ε Famz ; Table 2 ) based on the relative rates of carbon fixation associated with each respective metabolism. We included averaged depth-integrated carbon fixation rates of anammox [46] , [47] , [48] , [49] , [50] ; aerobic NH 4 + oxidation [55] and low-light-adapted cyanobacteria [93] , and min/max rates of sulfide oxidation [39] (i.e. corresponding to low/high SDAD scenarios, respectively). Depth integrated NH 4 + oxidation rates were estimated from discrete carbon fixation rates off northern Chile by Molina & Farías [55] , assuming nitrifying bacteria/archaea to be limited to ~100 m of the lower oxycline and upper OMZ. Sulfate-reducing bacteria in the ETSP are thought to be predominantly heterotrophic and provide a significant source of mineralized NH 4 + for anammox bacteria [13] , but are not expected to be a significant source of fixed carbon and are thereby not included in this calculation.